Development of an ultra-thin film comprised of a graphene membrane and carbon nanotube vein support Graphene, exhibiting superior mechanical, thermal, optical and electronic properties, has attracted great interest. Considering it being one-atom-thick, and the reduced mechanical strength at grain boundaries, the fabrication of large-area suspended chemical vapour deposition graphene remains a challenge. Here we report the fabrication of an ultra-thin free-standing carbon nanotube/graphene hybrid film, inspired by the vein–membrane structure found in nature. Such a square-centimetre-sized hybrid film can realize the overlaying of large-area single-layer chemical vapour deposition graphene on to a porous vein-like carbon nanotube network. The vein–membrane-like hybrid film, with graphene suspended on the carbon nanotube meshes, possesses excellent mechanical performance, optical transparency and good electrical conductivity. The ultra-thin hybrid film features an electron transparency close to 90%, which makes it an ideal gate electrode in vacuum electronics and a high-performance sample support in transmission electron microscopy. Graphene, as verified to be one-atom-thick by transmission electron microscopy (TEM) [1] , [2] , has attracted great interest because of its unique properties and potential applications [3] , [4] , [5] , [6] , [7] . Chemical vapour deposition (CVD) provides a promising way to synthesize large-area high-quality single-layer graphene [8] , [9] . However, owing to the severly weakened mechanical strength induced by its polycrystalline nature [10] , large-area (>1 mm 2 ) suspended graphene still cannot be easily achieved. Therefore, present research still focuses on the graphene with substrates (such as graphene on silicon wafers), despite the fact that the existence of the substrate would influence the properties of graphene and limit its applications [11] , [12] . To this end, the facile fabrication of large-area suspended graphene would be of both scientific and technological importance. Inspired by the macroscopic vein–membrane structure, we demonstrate an ultra-thin hybrid film comprised of a graphene membrane and a vein-like carbon nanotube network (CNT network). In nature, the vein–membrane structure (of the leaf and the insect wing, for example) is a kind of light-weight and mechanically robust structures (or morphologies) with specific functionalities, which has been widely mimicked in architectural vaults and other man-made macroscopic structures [13] , [14] . In our experiment, large-area single-layer CVD graphene is overlaid on to the porous vein-like CNT network, resulting in a free-standing ultra-thin hybrid film with a size up to square centimetres. Such a CNT/graphene hybrid film (CGF) realizes the suspending of graphene on CNT meshes, and shows an improved mechanical strength and electrical conductivity over the CNT network. Furthermore, the CGF features a very high electron transparency close to 90%. We demonstrate that the CGF can thus be used as a gate electrode in vacuum electronic devices and as a high-performance sample support in TEM. Fabrication of the CGF The fabrication process of the CGF is shown in Fig. 1 . Single-layer graphene was synthesized by CVD on Cu foils. Because graphene has been grown on both sides of the Cu foil ( Fig. 1a ), we have adopted an oxygen reactive-ion etching (RIE) process to remove graphene from one side (bottom) of the foil ( Fig. 1b ). Then, two layers of super-aligned CNT (SACNT) films [15] , [16] (see Methods and Supplementary Fig. S1 ) were cross-stacked on top of the graphene, after that alcohol treatment was used to make the CNT film (or CNT network, similar hereinafter) stick to the graphene ( Fig. 1c ) [16] . The CNT network is hoped to serve as a porous vein-like support during the fabrication process. The same chemical composition and bond structure of the CNT and graphene can ensure a strong adhesion between them, resulting in improved robustness of the CGF. Damage of the CGF, caused by the surface tension of the aqueous solution during the fabrication process, can thus be alleviated. After etching the Cu foil away, a free-standing CGF can be obtained ( Fig. 1d ). 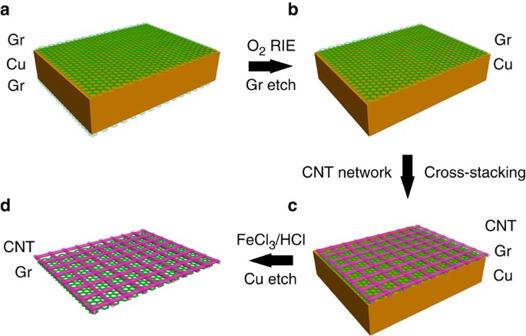Figure 1: Fabrication of CGFs. (a) Cu foil with graphene (Gr) on both sides after CVD growth. (b) Cu foil with only one side of graphene after oxygen RIE. (c) Graphene/Cu foil cross-stacked by CNT networks, and then infiltrated by alcohol. (d) CGF with a highly ordered layer-to-layer graphene/CNT network stacking structure, after etching the Cu foil with FeCl3/HCl solution. Figure 1: Fabrication of CGFs. ( a ) Cu foil with graphene (Gr) on both sides after CVD growth. ( b ) Cu foil with only one side of graphene after oxygen RIE. ( c ) Graphene/Cu foil cross-stacked by CNT networks, and then infiltrated by alcohol. ( d ) CGF with a highly ordered layer-to-layer graphene/CNT network stacking structure, after etching the Cu foil with FeCl 3 /HCl solution. Full size image By cross-stacking more layers of SACNT films or stretching the SACNT films before stacking, we can change the size of the CNT mesh to tune the size of individual suspended graphene ( Supplementary Fig. S2 ) [17] , [18] . The sizes of suspended graphene in the CGF with two-layer and eight-layer SACNT films are about 1 μm ( Supplementary Fig. S2a ) and 100–200 nm ( Supplementary Fig. S2b ), respectively. By replacing Cu foils with Ni foils during the CVD growth of graphene, we can also fabricate CGFs with multi-layer graphene. And by stacking two or more CGFs together in a certain order, CGFs with CNT/graphene/CNT, graphene/CNT/graphene stacking structures or more complex stacking structures can also be obtained. 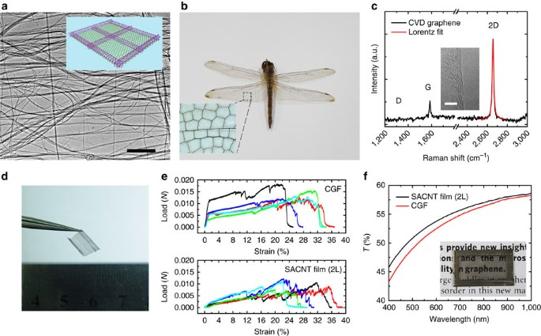Figure 2: Physical characterizations of CGFs. (a) TEM image and schematic illustration (inset ina) of the CGF. Scale bar, 1 μm. (b) Photograph of a dragonfly, whose wings have a vein–membrane structure, as indicated by the microscope photograph inset inb. (c) Raman spectrum of CVD graphene on Cu foil with laser energy of 1.96 eV, and the background signal of Cu foil is subtracted. The inset is a TEM image of the CVD graphene edge; scale bar, 5 nm. (d) A CGF (10 mm × 10 mm sized) handled by a tweezer, indicating its free-standing feature. (e) Load–strain curves of five CGFs and five two-layer (2L) SACNT films, both with a 45° angle between the tensile direction and the CNT aligned directions. The sizes of the CGF and SACNT film for the mechanical test are both 10 mm (L) × 5 mm (W). (f) Optical transmittance of the CGF and SACNT film. The inset shows the photograph of a CGF suspended on a stainless steel frame. Characterizations of the CGF Figure 2a shows a typical TEM image of the CGF with a vein–membrane-like structure formed by the CNT network and graphene (inset of Fig. 2a ), which is similar to the wing of dragonfly ( Fig. 2b ) in structure. Raman spectroscopy of as-grown CVD graphene on Cu foils ( Fig. 2c ) together with other characterization methods was used to confirm the single-layer feature of the graphene used in the CGF. Three Raman peaks are marked in Fig. 2c , including D peak (~1,350 cm −1 ), G peak (~1,585 cm −1 ) and 2D peak (~2,656 cm −1 ). No obvious D peak was found, indicating the defect-free feature in the signal collection spot [19] . The peak intensity ratio I 2D /I G ~5 feature suggests that the number of graphene layers is <3 (refs 8 , 19 , 20 ). In addition, with the single Lorentzian profile (with an 18 cm −1 linewidth) fitting of the 2D peak, the Raman characterization can attest that it is a single-layer graphene or a turbostratic (that is, not AB-stacking order) bilayer graphene with a rotational angle larger than 13° (refs 19 , 21 ). Considering the scanning electron microscopy image of graphene on Cu foil ( Supplementary Fig. S3a , providing information about the sample uniformity), the TEM image of the graphene edge (inset of Fig. 2c , showing a typical single-layer graphene feature) and the electron diffraction pattern of the sample ( Supplementary Fig. S3b ), we can conclude that it is a single-layer graphene. As single-layer graphene is only one-atom-thick [5] , [7] , the thickness of the CGF can be regarded as equal to that of the SACNT film (that is, tens of nanometres [16] ). The ultra-thin CGF is free-standing and can be easily handled by tweezers ( Fig. 2d ). It can be attached to various target substrates, such as stainless steel frames or conventional TEM grids according to different applications. The size of the CGF in our experiment is about 1–10 cm 2 . Larger area CGFs can also be fabricated in the same process due to the successful large-area synthesis of the CVD graphene [9] and the SACNT film [16] . Figure 2: Physical characterizations of CGFs. ( a ) TEM image and schematic illustration (inset in a ) of the CGF. Scale bar, 1 μm. ( b ) Photograph of a dragonfly, whose wings have a vein–membrane structure, as indicated by the microscope photograph inset in b . ( c ) Raman spectrum of CVD graphene on Cu foil with laser energy of 1.96 eV, and the background signal of Cu foil is subtracted. The inset is a TEM image of the CVD graphene edge; scale bar, 5 nm. ( d ) A CGF (10 mm × 10 mm sized) handled by a tweezer, indicating its free-standing feature. ( e ) Load–strain curves of five CGFs and five two-layer (2L) SACNT films, both with a 45° angle between the tensile direction and the CNT aligned directions. The sizes of the CGF and SACNT film for the mechanical test are both 10 mm (L) × 5 mm (W). ( f ) Optical transmittance of the CGF and SACNT film. The inset shows the photograph of a CGF suspended on a stainless steel frame. Full size image Such a free-standing CGF possesses some special features originating from its structure and the parent materials (that is, the CNT film and graphene). Compared with the parent two-layer (2L) SACNT film, the CGF shows a different and improved mechanical performance ( Fig. 2e ). They both show an elastic feature under strains smaller than ~2% and a plastic feature under strains from ~2 to ~30% before they are broken. At the strain of 30%, the in-plane Poisson’s ratio of the middle part of the film can be calculated as large as 2.86 ( Supplementary Fig. S4 ). With the existence of one-atom-thick graphene, the CGF can sustain a larger maximum load over the SACNT film (14.24±2.47 mN and 9.42±2.22 mN for CGFs and SACNT films, respectively). Although, no obvious difference in fracture strains (31.33±4.72% and 32.38±4.29% for CGFs and SACNT films, respectively) was found. Most importantly, the CGF shows a different mechanical feature from the SACNT film at the elastic region. The yield strains (that is, the critical strain where the sample becomes plastic) are 0.91±0.13% and 1.58±0.51% for CGFs and SACNT films, respectively. The yield loads are 5.87±2.77 mN and 1.26±0.48 mN for CGFs and SACNT films, respectively. As a result, Young’s modulus of the CGF can be calculated to be 2.34±0.89 GPa, which is an order larger than that of the SACNT film (0.35±0.21 GPa). These features mentioned above indicate that the overlaying of sub-nanometre-thick single-layer CVD graphene on the tens-of-nanometres-thick CNT film makes the film much stiffer at the elastic region and stronger on the whole. Such stiffer and stronger features can be interpreted as the hampered deformability and the reinforcement induced by the overlaid graphene membrane on the vein-like CNT network. As illustrated in Fig. 2a , the CGF includes large-area graphene adhered to SACNT film via strong van der Waals interactions. Compared with the parent SACNT film with network structure, the existence of graphene can reinforce the film and impede the deformation of the CNT network. Furthermore, previous experimental study of micron-sized single-layer CVD graphene (with a suspended size of about 2 μm in diameter) indicates that CVD graphene features a yield strain ~1.6% and Young’s modulus ~540±33 GPa [22] . On the basis of these results, we can predict a 14.7 mN equivalent yield load for the case of a 5-mm wide CVD graphene. Such a value is in agreement with the reinforcement induced by CVD graphene in the CGF, and its comparison with the yield loads of the CGF (5.87±2.77 mN) and the SACNT film (1.26±0.48 mN) also verifies the merits of the CNT network as a support to preserve the excellent mechanical performance of CVD graphene on the macroscopic scale. We also measured the optical transmittance and the sheet resistance of the CGF, and both of the results agree with the nature of CNT/graphene stacking structure. As reported in previous experimental work, single-layer graphene exhibits a practically wavelength-independent optical transmittance of 97.7% for an optical wavelength >500 nm [23] . Here we show that the overlaying of graphene causes a small transmittance decrease from the CNT network, from 53.7 to 52.5% at 600 nm ( Fig. 2f ), in agreement with the CNT/graphene stacking structure of the CGF. The sheet resistance of the CGF is 573 Ω −1 , which is smaller than those of SACNT films (~975 Ω −1 ) and single-layer CVD graphene (~887 Ω −1 , for the CVD graphene we used), also agrees with the stacking structure. By further doping the graphene, the sheet resistance of the film can be greatly decreased [9] , which holds out the possibility to use it as an ultra-thin, free-standing and flexible transparent conductive film [9] , [16] . Electron transparency of the CGF and corresponding applications Such a vein–membrane like CGF is of fairly high electron transparency. The electron transparency was measured in an ultrahigh vacuum system ( Fig. 3a , see Methods for details). Electron beams (e-beams) from the cathode (a thermionic electron gun) were focused to pass through the CGF only, so that the electron transparency can be calculated from currents of the CGF and anode. Fig. 3b shows the measured electron transparency of the CGF, which increases with the incident electron energy. The transparency can be as high as 90% when the energy is above 1 keV. 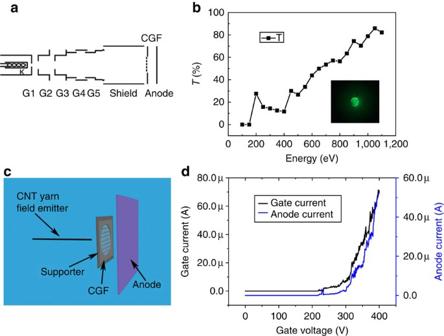Figure 3: Electron transparency and field emission gate electrode test of CGFs. (a) Schematic illustration of the electron transparency measurement system. (b) Electron transparency of the CGF. The inset shows the anode image during the measurement. (c) Schematic illustration of a field emission system with a CGF as the gate electrode, and a CNT yarn emitter. (d) The dependences of anode and gate currents with various gate voltages, the anode voltage was fixed at 1,100 V. The ratio of anode current/total current is lower than 90%, because the e-beam is not focused and some of them have been collected by the supporter inc. Figure 3: Electron transparency and field emission gate electrode test of CGFs. ( a ) Schematic illustration of the electron transparency measurement system. ( b ) Electron transparency of the CGF. The inset shows the anode image during the measurement. ( c ) Schematic illustration of a field emission system with a CGF as the gate electrode, and a CNT yarn emitter. ( d ) The dependences of anode and gate currents with various gate voltages, the anode voltage was fixed at 1,100 V. The ratio of anode current/total current is lower than 90%, because the e-beam is not focused and some of them have been collected by the supporter in c . Full size image We then applied the electron transparent CGF as a gate electrode—a necessary component to control the current in vacuum electronic devices. A gate electrode with high electron transparency would improve the performance of the vacuum electronic devices, such as triode tubes, microwave tubes [24] , ionization vacuum gauges and gas electron multipiers [25] , [26] , by improving the amplification factor and lowering the power consumption [27] , [28] , [29] . Indeed, high electron transparency gate electrode is a desired component in vacuum electronics. Traditional gate electrodes are grids woven with metal wires, or fabricated by lithography. They can also realize 90% or above electron transparency. However, attempts to improve the transparency of these gate electrodes, by increasing the mesh size, often result in poor electric field uniformity, which instead deteriorates the devices’ performance [24] . The electron transparent CGF would be able to solve this problem: the membrane structure of the CGF ( Fig. 2a ) makes the gate electrode similar to a planar electrode, therefore, would be able to guarantee better electrical field uniformity. The mechanical strength of the CGF can also contribute to its manipulation and integration in corresponding devices. As an example, we have applied the CGF as a gate electrode in a CNT yarn field emission system ( Fig. 3c , see Methods for details). Figure 3d shows the gate voltage dependence of the anode and gate currents, with an anode voltage fixed at 1,100 V. It can be seen that the CGF gate can control the anode current very effectively. The field enhancement factor of the CNT yarn emitter in the CGF gate field emission experiment was calculated to be as large as that of the field emission system with a metal plate as the gate (~5 × 10 4 ) [30] . The calculation was based on the Fowler–Nordheim field emission theory [31] : where j 0 is the emission current density of the emitter, ϕ is the work function of the emitter (~4.6 eV for the CNT yarn [32] ), E is the electric field intensity of the emitter ( E=γU/d , γ is the field enhancement factor, U is the gate voltage, d is the distance between CNT yarn emitter and the CGF gate) and θ is the so-called Nordheim function, which is usually viewed as 1. Considering that the field enhancement factor of the CNT yarn emitter is about 5 × 10 4 , the applied voltage ( U ) during the emission is about 200–400 V and that the distance between the emitter and the gate ( d ) is 2 mm in our experiment, the corresponding electric field intensity of the emitter can be worked out to be about 5–10 V nm −1 . Further integration of the CGF in vacuum microelectronics devices would enable good control of the emission and can optimize the performance, owing to its ability to guarantee the electric field uniformity. Besides the use as gate electrodes, the CGF can be used as an easy-made large-area and high-performance TEM sample support, which also requires a high electron transparency. As has been reported, one-atom-thick graphene is an excellent candidate for TEM supports owing to its crystalline structure, high electrical conductivity, very low background noise, and most importantly high electron transparency [1] , [2] , [33] . CVD graphene TEM supports [34] , [35] can successfully meet the demand of batch applications, but previous methods may induce polymer contamination [36] , and the photolithography involved fabrication process is complicated. Facilely, CGF TEM grids can be achieved by choosing conventional Cu TEM grids as the target substrate in the fabrication process. The membrane structure and the high electron transparency result in a CGF grid possessing larger effective areas to support samples and a lower background noise, than our previous CNT film grids [37] and graphene oxide–CNT grids [38] . The carbon-only composition of the CGF would be also helpful for chemical composition analysis of samples ( Supplementary Fig. S5 ), and the high mechanical performance can ensure the durability of the grid. At the same time, the network of CNT in the CGF can confine damage of the graphene during sample preparations and TEM observations ( Fig. 4c ), which is of practical importance. Owing to the existence of the graphene support ( Fig. 4a,b ), the observation of an ensemble of nano materials, such as Au nanoparticles (NPs), at the same time becomes possible ( Fig. 5 ). The arrangement, sizes and the crystalline structures of Au NPs could be clearly seen ( Fig. 5a,b ). Furthermore, owing to the stability of the graphene membrane guaranteed by the vein-like CNT network, the CGF grid is very suitable for observations of NPs’ evolution under high-resolution TEM (HRTEM). The crystalline structure evolution of individual Au NPs (The circles marked as 1 in Fig. 5c,d , originating from the lattice mismatch between graphene and Au NPs [39] .) and the interactions among them (such as the NPs’ coalescence [38] , [39] , the boxes marked as 2 in Fig. 5c,d ) under e-beam irradiation were observed. Both the crystalline structure evolution and coalescence of the Au NPs were found to speed up under a higher acceleration voltage ( Fig. 6 ). Besides, owing to the e-beam irradiation, graphene began to be destroyed and the distances between two NPs were shortened at the same time. As a result, many NPs finally merged together and formed a bigger NP ( Fig. 6c ). These results imply that e-beam irradiation would contribute to the coalescence and crystalline structure evolution of NPs. It also implies the possibility to study chemical reactions (such as the nanocrystal growth) under TEM using the CGF grid, which should be of scientific importance [40] . 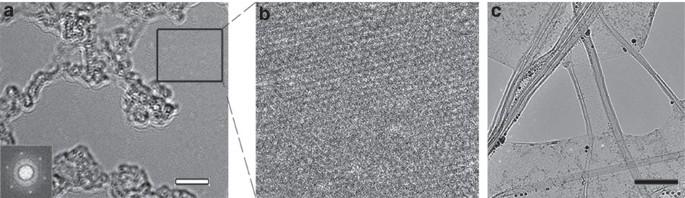Figure 4: HRTEM images of CGFs. (a) HRTEM image of suspended graphene in the CGF. The inset shows the fast Fourier transform result. Some amorphous adsorbates on graphene can been seen as has also been reported previously in refs1,2,34. Scale bar, 5 nm. (b) Local magnification of the marked zone ina. (c) CGF with partly damaged graphene, after placing Au NPs (the black balls in the TEM image) on it. Scale bar, 100 nm. Figure 4: HRTEM images of CGFs. ( a ) HRTEM image of suspended graphene in the CGF. The inset shows the fast Fourier transform result. Some amorphous adsorbates on graphene can been seen as has also been reported previously in refs 1 , 2 , 34 . Scale bar, 5 nm. ( b ) Local magnification of the marked zone in a . ( c ) CGF with partly damaged graphene, after placing Au NPs (the black balls in the TEM image) on it. Scale bar, 100 nm. 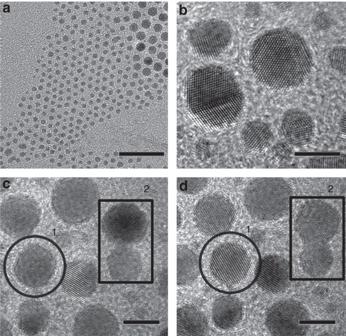Figure 5: HRTEM images of Au NPs on CGF TEM grids. (a,b) HRTEM images of monodispersed Au NPs/cyclohexane on CGF at different magnifications. (c,d) The evolution of monodispersed Au NPs/cyclohexane before (c) and after (d) a 10-s electron-beam (e-beam) irradiation. The circles marked as 1 incanddshow the crystalline structure evolution of individual Au NPs. The boxes marked as 2 incanddshow the coalescence of the Au NPs. The acceleration voltage was 200 kV. The scale bars inaandb–dare 25 nm and 5 nm, respectively. Full size image Figure 5: HRTEM images of Au NPs on CGF TEM grids. ( a , b ) HRTEM images of monodispersed Au NPs/cyclohexane on CGF at different magnifications. ( c , d ) The evolution of monodispersed Au NPs/cyclohexane before ( c ) and after ( d ) a 10-s electron-beam (e-beam) irradiation. The circles marked as 1 in c and d show the crystalline structure evolution of individual Au NPs. The boxes marked as 2 in c and d show the coalescence of the Au NPs. The acceleration voltage was 200 kV. The scale bars in a and b – d are 25 nm and 5 nm, respectively. 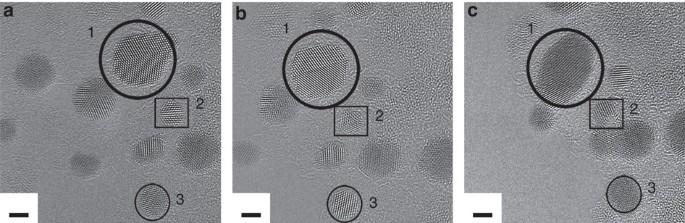Figure 6: Evolution of Au NPs on CGF TEM grid with higher voltage. (a) TEM image of Au NPs on CGF. (b) TEM image of Au NPs on CGF, after a 5 s e-beam irradiation. (c) TEM image of Au NPs on CGF, after a 10 s e-beam irradiation. Circles/boxes numbered 1–3 ina–cmark some Au NPs during the evolution and coalescence. All images were taken using a Titan G2 60–300 TEM, with a 300 kV acceleration voltage. The scale bars ina–care all 2 nm. Full size image Figure 6: Evolution of Au NPs on CGF TEM grid with higher voltage. ( a ) TEM image of Au NPs on CGF. ( b ) TEM image of Au NPs on CGF, after a 5 s e-beam irradiation. ( c ) TEM image of Au NPs on CGF, after a 10 s e-beam irradiation. Circles/boxes numbered 1–3 in a – c mark some Au NPs during the evolution and coalescence. All images were taken using a Titan G2 60–300 TEM, with a 300 kV acceleration voltage. The scale bars in a – c are all 2 nm. Full size image In conclusion, we have used the porous CNT network to support large-area single-layer CVD graphene and get an ultra-thin centimetre-sized free-standing vein–membrane-like CGF. The method is facile and scalable. The CGF, with graphene suspended on CNT meshes, exhibits some unique properties, such as excellent mechanical performance, optical transparency and good electrical conductivity. Owing to its nearly 90% electron transparency and excellent mechanical performance, the hybrid film can be used as an ideal gate electrode for vacuum electronics and an easy-made large-area high-performance sample support in TEM. Furthermore, the simple fabrication method, the mimetic structure, the unique properties and the existence of suspended graphene, will enable more fundamental research and real applications of the CGF in the near future. Fabrication of CGFs CVD graphene was synthesized on Cu foils (Alfa Aesar, item no. 13382) in a fused silica tube (22 mm inner diameter) with a hot-wall furnace (Lindberg Blue M TF55035C-1). The CVD growth parameters were similar to those in ref. 8 : The Cu foil were annealed in hydrogen atmosphere (2 standard cubic centimeter per minute (sccm), 40 mTorr, 1000 °C, 40 min), before the graphene growth process (2 sccm hydrogen and 35 sccm methane, 500 mTorr, 1,000 °C, 20 min). RIE treatment (40 sccm oxygen, 10 Pa, 20 W, 10 s) was carried out with an Anelva L-451D-L Etching System. The SACNT film was drawn from the SACNT array, with CNTs aligned in the drawing direction [16] . CNT film/graphene/Cu foil was floated on the ferric chloride aqueous solution (0.5 mol l −1 , with dilute hydrochloric acid) for 2 h to etch the Cu foil. Physical characterization The structure of the CGF was characterized by Raman spectroscopy (Jobin Yvon LabRAM HR800) and TEM (FEI Tecnai G2 F20 S-Twin TEM). For TEM characterization of the CGF and Au NPs on it, the acceleration voltages were 120 and 200 kV, respectively. Au NPs were placed on the CGF by a method similar to our previous work (by dropping a drop of Au NPs/cyclohexane on the TEM grid) [37] , [38] . The optical transmittance and the mechanical property of the film were measured with a PerkinElmer-Lambda 950 (ultraviolet–visible–near-infrared) Spectrometer and an Instron 5848 MicroTester, respectively. Electron transparency test The electron transparency of CGF was tested in a vacuum chamber with a base pressure of 7 × 10 −6 Pa. A thermionic electron gun ( Fig. 3a ) was used as the electron source. The heating voltage of the filament is 12 V. The cathode was kept at 10 V. G1 was kept at ground voltage. G2 and G4 were kept at 300 V to focus the electron spot to fit the sample size. G3, G5 and the shield were set to the same voltage as the sample. The anode voltage was 20 V higher than the sample, which was enough to collect the transmitted electrons. The transparency was calculated based on the current collected by the CGF and anode. CGF gate electrode test The test of CGF field emission gate was carried out with a field emitter (a SACNT yarn, diameter about 10 μm) in a vacuum chamber of a base pressure 5 × 10 −5 Pa. The CGF was placed on metal supporter with a hole of 5 mm diameter. The anode was a phosphor-coated transparent indium tin oxide glass. The distance between the emitter tip and the CGF gate was about 2 mm, and distance between the CGF and the anode was about 10 mm. The current–voltage (I–V) measurements of the gate and anode were performed with two Keithley 2410 source measurement units. How to cite this article: Lin, X. et al . Development of an ultra-thin film comprised of a graphene membrane and carbon nanotube vein support. Nat. Commun. 4:2920 doi: 10.1038/ncomms3920 (2013).